Stimuli-sensitive intrinsically disordered protein brushes Grafting polymers onto surfaces at high density to yield polymer brush coatings is a widely employed strategy to reduce biofouling and interfacial friction. These brushes almost universally feature synthetic polymers, which are often heterogeneous and do not readily allow incorporation of chemical functionalities at precise sites along the constituent chains. To complement these synthetic systems, we introduce a biomimetic, recombinant intrinsically disordered protein that can assemble into an environment-sensitive brush. This macromolecule adopts an extended conformation and can be grafted to solid supports to form oriented protein brushes that swell and collapse dramatically with changes in solution pH and ionic strength. We illustrate the value of sequence specificity by using proteases with mutually orthogonal recognition sites to modulate brush height in situ to predictable values. This study demonstrates that stimuli-responsive brushes can be fabricated from proteins and introduces them as a new class of smart biomaterial building blocks. Polymer brushes form when macromolecular chains are end-tethered to surfaces at high grafting densities [1] , [2] . The swelling and mutual steric repulsion of the polymers cause the chains to stretch and extend into the solvent, producing a molecular coating that can reduce non-specific interactions of the underlying surface with cells and biological macromolecules [3] . Some polymer brushes are environment-sensitive, with specific changes in solvent conditions triggering their expansion or collapse. These materials can be used to exert dynamic control over the spatial presentation of regulatory peptides and are under investigation for many applications [4] , [5] , including sensors [6] , flow valves [7] and controlled drug release systems [8] . However, because these brushes are almost universally constructed from synthetic polymers, they are frequently somewhat heterogeneous and are challenging to modify at specific monomeric positions along the chain. [9] , [10] While there have been notable successes integrating these materials with proteins to control biological function [11] , [12] , such strategies require covalent conjugation of the protein to the polymer, which can be inefficient and can compromise biological function [13] . These limitations can potentially be overcome by creating a new class of polymer brushes based on intrinsically disordered proteins (IDPs). IDPs are attractive candidates for fabricating polymer brushes primarily because they lack secondary structure and adopt an extended conformation. For example, these properties of IDPs were recently harnessed to design an ‘entropic bristle’ based fusion tag for solubilizing recalcitrant recombinant proteins [14] . Furthermore, IDPs can also be designed and purified to near-perfect homogeneity, with the naturally occurring amino acids providing a chemically diverse palette for the control of chain properties such as charge distribution and hydrophobicity. In addition, the potential to synthesize proteins with either bioactive epitopes fused to IDP segments or sequences that can be enzymatically modified with high specificity provides an elegant way to create biofunctional interfaces. Here we create a stimuli-responsive IDP that can be assembled onto a surface as a polymer brush. We base our design on the disordered C-terminal sidearm domain of the heavy subunit of the neurofilament complex (NF-H), which is believed to function as an entropic spring that facilitates the assembly, mechanics and transport of neurofilaments (NFs) in the neuronal cytoskeleton [15] . This subunit has two notable features: first, it contains a large and nearly equal number of cationic (Lys, Arg) and anionic (Glu, Asp) residues, rendering it highly charged locally but nominally neutral globally. Second, it consists of a series of Lys–Ser–Pro (KSP) motifs, which allows for the modulation of protein charge in vivo via phosphorylation of the Ser residues. We show that this engineered protein (rNFH-SA) adopts an extended, disordered conformation in solution and can be grafted in an oriented manner to solid supports to yield IDP brushes that swell and collapse in response to changes in solution pH and ionic strength. We also show that the heights of these brushes may be modulated through the application of proteases that recognize specific sequences within the brush. Purification and characterization of rNFH-SA We engineered a protein construct, rNFH-SA, containing residues 426–1066 from the rat NF-H sidearm domain, flanked by an N-terminal tetra-Cys tag to permit oriented assembly onto thiol-reactive surfaces and a C-terminal poly-His-Asn tag (HN tag) to facilitate purification ( Fig. 1a ; see Methods and Supplementary Fig. 1 for details of cloning, expression and purification). The circular dichroism (CD) spectrum of rNFH-SA ( Fig. 1b ) was consistent with that of an IDP, characterized by a minimum centred at ~200 nm with negligible contribution from secondary structure-forming elements [16] . Dynamic light scattering measurements yielded a hydrodynamic radius ( r H ) of 10 nm, significantly larger than the expected radius of globular proteins ( r H ≈4 nm) of similar molecular weight [17] , indicating that the protein adopts an extended conformation ( Fig. 1c , Supplementary Note 1 , Supplementary Fig. 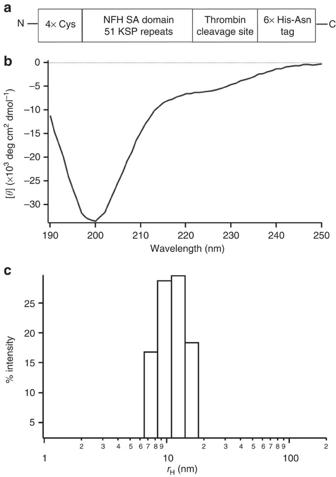Figure 1: Characterization of rNFH-SA. (a) Domain structure of rNFH-SA showing the N-terminal tetra-Cys tag, the IDP domain and the C-terminal HN tag. The NF-H sidearm sequence lacks native cysteines, thereby allowing the use of the tetra-Cys tag for oriented assembly. (b) Far-ultraviolet CD spectrum of rNFH-SA. (c) Distribution of hydrodynamic radii (rH) obtained from dynamic light scattering. 2 and Supplementary Table 1 ) [18] . Figure 1: Characterization of rNFH-SA. ( a ) Domain structure of rNFH-SA showing the N-terminal tetra-Cys tag, the IDP domain and the C-terminal HN tag. The NF-H sidearm sequence lacks native cysteines, thereby allowing the use of the tetra-Cys tag for oriented assembly. ( b ) Far-ultraviolet CD spectrum of rNFH-SA. ( c ) Distribution of hydrodynamic radii ( r H ) obtained from dynamic light scattering. Full size image Brush formation by surface immobilized rNFH-SA To determine if rNFH-SA could be assembled into a polymer brush, we monitored the immobilization of the protein on maleimide-functionalized substrates (see Supplementary Fig. 3 ) using quartz crystal microbalance with dissipation (QCM-D). The adsorption of rNFH-SA was registered as a decrease in the normalized frequency ( Δf/n ) and an increase in the dissipation ( ΔD ). Using a protein concentration of ~0.5 mg ml −1 , we were able to capture the transition of the bound protein layer from a collapsed ‘mushroom’ to an extended ‘brush’ configuration ( Fig. 2a,b ). The marked change in Δf/n and ΔD ( Fig. 2a ) within the first 5–10 min indicates rapid immobilization of the protein on the surface. After ~20 min, the change in Δf/n and ΔD was much slower, suggesting that the chains initially grafted to the surface were hindering additional protein molecules from tethering. After considerable time had elapsed (~100 min), Δf/n decreased further, accompanied by an increase in ΔD . This observation suggests that the bound protein molecules had swollen into an extended conformation, thereby allowing access to new binding sites on the surface and accelerating the tethering of additional protein molecules as has been observed previously [19] , [20] . This mushroom-to-brush transition is also evident from the plot of ΔD versus − Δf/n ( Fig. 2b ), which shows that the increase in the protein-grafting rate is accompanied by a change in the structure of the surface layer. In the brush regime, each newly immobilized protein chain causes a comparatively greater increase in dissipation (observed as an increase in slope of the plot), as would be expected for an extended molecule. To achieve maximum surface coverage, the substrate was incubated with a highly concentrated protein solution (~5 mg ml −1 ) for ~20 h. The time-dependent change in Δf/n and ΔD was monitored and the hydrated adsorbed mass per unit area was calculated (37.4 ng mm −2 ) by fitting the data to the Voigt–Voinova viscoelastic layer model ( Supplementary Fig. 4 ) [21] . To obtain a true measure of the surface density without the confounding effects of brush hydration and swelling, spectroscopic ellipsometry measurements were performed on a dry surface prepared under conditions identical to the latter QCM-D measurements. The calculated surface density ( Supplementary Note 2 ) of 0.02 molecules per nm 2 corresponds to an intermolecular spacing of 7.75 nm (assuming a hexagonal close packing arrangement) and indicates that protein brush layers were formed ( Supplementary Note 3 ). These conditions were used to generate protein-tethered surfaces for all subsequent studies, and the ellipsometric grafting density was used in subsequent analyses. 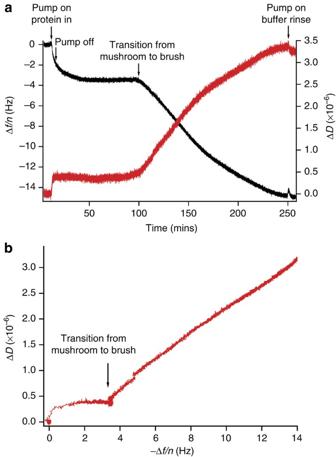Figure 2: Brush formation observed by QCM-D measurements. (a)Δf/n(black) andΔD(red) for the overtonen=3 as a function of time obtained by QCM-D experiments. A protein concentration of 0.5 mg ml−1was used to capture the transition from a collapsed ‘mushroom’ to an extended ‘brush’ regime. The protein solution was allowed to enter the chamber containing the functionalized sensor and subsequently allowed to stand in the chamber for ~4 h. Finally, buffer was introduced into the chamber to wash away unbound protein. (b)ΔDversus −Δf/ntrace showing a sharp change in trend at ~100 min. A steep slope at later time points indicates that the thickness increases significantly with grafting density and that the chains adopt an extended conformation. Figure 2: Brush formation observed by QCM-D measurements. ( a ) Δf/n (black) and ΔD (red) for the overtone n =3 as a function of time obtained by QCM-D experiments. A protein concentration of 0.5 mg ml −1 was used to capture the transition from a collapsed ‘mushroom’ to an extended ‘brush’ regime. The protein solution was allowed to enter the chamber containing the functionalized sensor and subsequently allowed to stand in the chamber for ~4 h. Finally, buffer was introduced into the chamber to wash away unbound protein. ( b ) ΔD versus − Δf/n trace showing a sharp change in trend at ~100 min. A steep slope at later time points indicates that the thickness increases significantly with grafting density and that the chains adopt an extended conformation. Full size image To further quantify and characterize the bound layer of rNFH-SA, we used atomic force microscopy (AFM) to measure forces exerted by the immobilized IDP layer ( Fig. 3 ). The experiments were performed at pH 2.4 and 10.9 to encompass the nominal p K a values of glutamate and lysine, and render rNFH-SA highly positively or negatively charged, respectively. We observed strong tip–sample repulsive forces from rNFH-SA layers at separation distances much greater than the Debye length ( Supplementary Fig. 5 ). The long-range repulsive forces measured on rNFH-SA surfaces, in comparison to Cys-immobilized surfaces ( Fig. 3 ), indicate the presence of a brush layer and are consistent with the QCM-D and ellipsometry data. 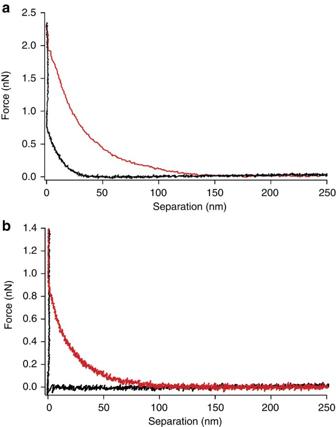Figure 3: Comparison of force curves. AFM force–distance curves measured with either rNFH-SA (red) or Cys (black) immobilized on the maleimide-functionalized glass surface at (a) pH 10.9, 2 mM ionic strength and (b) pH 2.4, 4 mM ionic strength. The conditions represented here show maximum brush heights. Long-range forces are observed only in the case of protein-tethered surfaces. Figure 3: Comparison of force curves. AFM force–distance curves measured with either rNFH-SA (red) or Cys (black) immobilized on the maleimide-functionalized glass surface at ( a ) pH 10.9, 2 mM ionic strength and ( b ) pH 2.4, 4 mM ionic strength. The conditions represented here show maximum brush heights. Long-range forces are observed only in the case of protein-tethered surfaces. Full size image Influence of ionic strength on the brush height To explore the properties of the IDP brush, AFM measurements were repeated over a range of ionic strengths ( I ) and the brush height was estimated as the tip–sample separation at which the force began to increase from zero ( Fig. 4 ). At both pH values, we observed a regime in which brush height decreased with increasing ionic strength ( I >2 mM for pH 10.9; the entire range for pH 2.4). These observations can be rationalized based on polyelectrolyte theory since the IDP behaves like a highly charged polymer under the chosen pH conditions. At I >2 mM, the protein brush is forced into the ‘salted brush’ regime due to the imbalance in the ionic strength inside and outside the brush. As the ionic strength increases, the charges on the chains are progressively screened, leading to a reduction in electrostatic repulsion and a decrease in brush height ( Supplementary Fig. 6 ). The experimental results ( Fig. 4 ) show a qualitative agreement with the mean-field theory of weak polyelectrolyte brushes ( Supplementary Note 4 and Supplementary Fig. 7 ) [22] , [23] , which predicts that the brush should collapse with increasing salt concentration ( C ), but only as a relatively weak power law ( C −1/3 ). We see a comparatively steeper ionic strength-dependence, which has been previously observed in synthetic polymer systems [24] , [25] , [26] , [27] , [28] , [29] and may arise from the local modulation of protein charge-based interactions due to added salt. 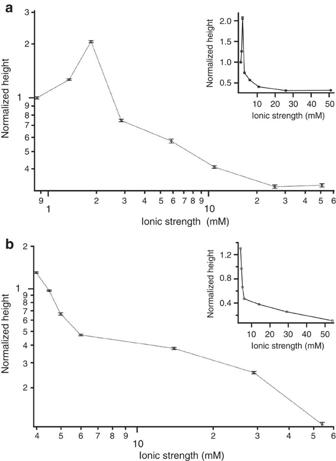Figure 4: Changes in brush height as a function of ionic strength. Brush heights were measured at (a) pH 10.9 and (b) pH 2.4. To account for potential sample-to-sample variations, data values are normalized to the brush height measured at pH 10.9, 0 mM NaCl for the corresponding surface (57±4 nm). The insets depict the same data plotted on linear scales. Error bars indicate s.e. of the normalized brush height calculated for 400–800 force curves sampled at different points on the surface. Figure 4: Changes in brush height as a function of ionic strength. Brush heights were measured at ( a ) pH 10.9 and ( b ) pH 2.4. To account for potential sample-to-sample variations, data values are normalized to the brush height measured at pH 10.9, 0 mM NaCl for the corresponding surface (57±4 nm). The insets depict the same data plotted on linear scales. Error bars indicate s.e. of the normalized brush height calculated for 400–800 force curves sampled at different points on the surface. Full size image At pH 10.9, below a critical ionic strength (~2 mM), the system enters an ‘osmotic brush’ regime in which the brush height increases with ionic strength. This phenomenon is based on a shift in the protonation/deprotonation equilibrium at low ionic strengths [24] . The local concentration of protons within the brush in the absence of salt is governed by the requirement of charge neutrality. However, when a small amount of salt is added, some of these cations can be exchanged with the protons inside the brush without affecting charge neutrality. As a consequence, the pH within the brush increases, thereby increasing the degree of deprotonation of the protein chains. This results in greater chain stretching due to counterion-induced osmotic swelling and increased inter- and intra-molecular electrostatic repulsion associated with chain ionization, as has been observed with synthetic polyelectrolyte and polyampholyte brush systems [24] , [28] , [29] . Above a critical ionic strength, this exchange mechanism saturates and the system enters the ‘salted brush’ regime, in which further addition of salt collapses the brush due to electrostatic screening ( Supplementary Figs 6 and 7 ). An analogous low-salt ‘osmotic brush’ regime was not observed at pH 2.4 due to the high baseline ionic strength. Importantly, this salt-responsiveness is consistent with recent theoretical/computational descriptions of native NF sidearm domains as polyelectrolyte brushes [30] , [31] , and the high-resolution structural characterization of NF networks [32] . However, the low-salt osmotic brush regime has not been reported previously for NF assemblies. Influence of pH on the brush height Next, we explored the possibility of pH-induced conformational changes in the rNFH-SA brushes ( Fig. 5 ). We chose a range of pH values that encompassed the nominal p K a of glutamate (4.1), the theoretical pI of the protein (6.3), and the nominal p K a of lysine (10.7). At pH>10.7, the carboxylate side chains are charged, while the lysine side chains remain largely neutral. Here polyelectrolyte effects dominate. As the pH is decreased, the lysine side chains are protonated, increasing the number of cationic residues along the polymer chain. Polyampholyte behaviour now dominates, with salt bridges forming between oppositely charged side chains along the length of the protein (or between protein chains in close proximity), resulting in a collapsed brush conformation. This behaviour continues through the minimum of the curve until the pI is reached. As the pH is reduced further, the carboxylate side chains become progressively protonated and thus neutral; simultaneously, the lysine side chains gain additional cationic character, and polyelectrolyte behaviour is again observed ( Supplementary Fig. 6 ). The expansion observed at the extremes are likely due to repulsive interactions between closely spaced like-charges [33] . These effects collectively produce a threefold variation in brush thickness over this pH range. Such pH-responsive thickness changes were recently reported in a more modest form (1.2–1.6-fold) for immobilized resilin-mimetic protein bilayers [34] . When the magnitude of the charge on the protein at various pH values ( Fig. 5 , broken line) is compared with the pH dependence of brush height, we observe that both curves follow a similar trend, attaining maxima of charge and height at either end of the pH spectrum. Interestingly, there is a slight pH offset between the two curves, which may be due to the fact that the theoretical charge curve assumes the nominal p K a values of the free amino acids. Comparison of the observed pH dependence with calculations based on the mean-field theory ( Supplementary Note 4 and Supplementary Fig. 8 ) suggests that the local chemical and electrostatic environment in the brush produces p K a shifts in some or all of the titratable residues, as observed in previous studies [35] . This pI-centred swelling behaviour has been previously observed for synthetic polyampholytes with charges randomly distributed along their length, which displayed at least threefold higher degree of swelling than mixed brushes of oppositely charged polyelectrolytes [36] , [37] . Recombinantly redistributing local charge density within rNFH-SA may offer additional opportunities to expand and tune these swelling dynamics [38] . 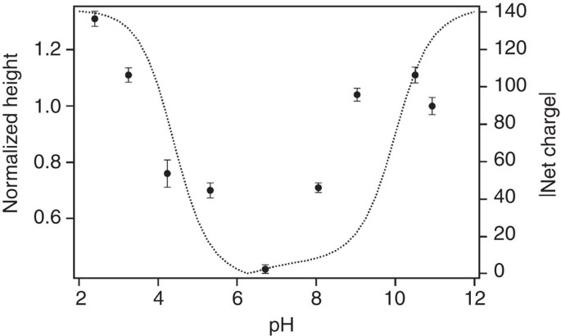Figure 5: Variations in brush height as a function of pH. Variations in brush height as a function of pH. Brush heights (closed circle) were measured with no additional salt added to the solution. All brush heights have been normalized to the value at pH 10.9, 0 mM NaCl. The absolute value of the charge on the protein (irrespective of the nature of charge) is shown as a broken line for comparison. Error bars indicate s.e. of the normalized brush height calculated for 400–800 force curves sampled at different points on the surface. Figure 5: Variations in brush height as a function of pH. Variations in brush height as a function of pH. Brush heights (closed circle) were measured with no additional salt added to the solution. All brush heights have been normalized to the value at pH 10.9, 0 mM NaCl. The absolute value of the charge on the protein (irrespective of the nature of charge) is shown as a broken line for comparison. Error bars indicate s.e. of the normalized brush height calculated for 400–800 force curves sampled at different points on the surface. Full size image In situ protease digestion of rNFH-SA brushes An additional and relatively unique feature of a protein-based brush is the ability to incorporate proteolytic cleavage sites into the polymer chain, which should in principle enable shortening or ‘shaving’ of the polymer brush with high precision upon addition of the cognate protease. To explore this concept, we assembled rNFH-SA brushes and applied one of two proteases: thrombin, a serine protease that cleaves rNFH-SA at a recognition site (LVPR|GS) located just ahead of the HN tag on the C terminus of the protein, and clostripain, an ArgC endoproteinase that cleaves at five sites along the length of the protein, the deepest of which is 253 residues from the top edge of the brush ( Fig. 6a ). A droplet of the protease was incubated with the rNFH-SA brush for a defined time before being washed off, and then the C-terminal HN tag was visualized by immunofluorescence ( Fig. 6b,c ). Both enzymes are capable of cleaving off the HN tag as evidenced by the loss of fluorescence in the region exposed to the protease; furthermore, enzymatic cleavage was reasonably well-contained within the droplet boundary, effectively patterning the brush height via confined proteolysis. By treating with the appropriate enzyme and measuring resulting changes in brush height by AFM, we found that we could specifically and spatially ‘shave’ the brush at the expected sites along the sequence ( Fig. 6d,e ). Specifically, addition of thrombin produced a loss of fluorescence (indicating successful enzymatic cleavage) without producing a significant change in brush height by AFM. Conversely, addition of clostripain produced the same loss of fluorescence while reducing brush height by 20%. Thus, brush height may be modulated in situ under physiological conditions to precise and predictable values by taking advantage of proteolytic cleavage sites, which in principle could be designed into the sequence a priori . 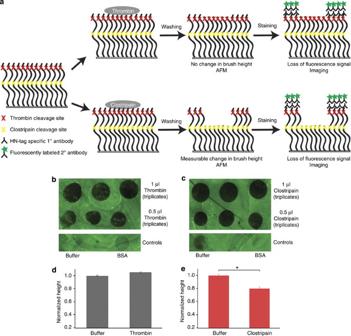Figure 6:In situprotease digestion of rNFH-SA brush. (a) Schematic representation of the protease digestion experiment. Digestion is accomplishedin situon immobilized rNFH-SA brush. The thrombin cleavage site (red cross) is very close to the surface (19 amino acids deep) while the deepest clostripain digestion site (yellow cross) is 253 amino acids from the top edge of the brush. Although both enzymes cleave off the HN tag leading to a loss of immunofluorescence, only clostripain digestion produces a measurable change in the brush height. Fluorescence image of the protein brushes digested with (b) thrombin and (c) clostripain. The clostripain buffer contains Ca2+, a divalent cation that could interact with the HN tag53,54,55; these interactions likely affect the accessibility of the HN-tag to the antibody, thereby causing a minor decrease in fluorescence. Comparison of normalized brush heights calculated from AFM experiments for (d) thrombin- and (e) clostripain-digested surfaces. Data represent mean±s.e. across ~1,000 force curves on a single surface; *P<0.01 by Student’st-test. The brush heights were normalized to the height measured for the corresponding buffer incubated surface (57±4 nm). Figure 6: In situ protease digestion of rNFH-SA brush. ( a ) Schematic representation of the protease digestion experiment. Digestion is accomplished in situ on immobilized rNFH-SA brush. The thrombin cleavage site (red cross) is very close to the surface (19 amino acids deep) while the deepest clostripain digestion site (yellow cross) is 253 amino acids from the top edge of the brush. Although both enzymes cleave off the HN tag leading to a loss of immunofluorescence, only clostripain digestion produces a measurable change in the brush height. Fluorescence image of the protein brushes digested with ( b ) thrombin and ( c ) clostripain. The clostripain buffer contains Ca 2+ , a divalent cation that could interact with the HN tag [53] , [54] , [55] ; these interactions likely affect the accessibility of the HN-tag to the antibody, thereby causing a minor decrease in fluorescence. Comparison of normalized brush heights calculated from AFM experiments for ( d ) thrombin- and ( e ) clostripain-digested surfaces. Data represent mean±s.e. across ~1,000 force curves on a single surface; * P <0.01 by Student’s t -test. The brush heights were normalized to the height measured for the corresponding buffer incubated surface (57±4 nm). Full size image To our knowledge, our study represents the first instance of a protein-based polymer brush system whose conformational properties can be strongly modulated by changes in pH and ionic strength. Notably, this material is recombinantly expressed, forms brushes, and yields a nearly six to tenfold dynamic range in brush thickness as ionic strength is varied and a threefold range as pH is varied. This dynamic range is comparable to many existing synthetic polymer brush systems and suggests that these materials may serve as an attractive complement or alternative to synthetic systems in specific settings [24] , [39] . It is also conceivable that this dynamic range could be shifted, widened, or narrowed in interesting ways by exerting more control over the grafting density, such as by using cloud point grafting to achieve very dense brushes [40] , [41] . Furthermore, we have demonstrated that we can use proteases to reduce the height of the brush in situ by cleaving the constituent chains at well-defined points. The extensive suite of proteases and protease recognition sites—any of which could be introduced into the sequence at one or more arbitrary positions—should provide a versatile toolbox for controlling IDP brush properties in a dynamic and specific manner. Analogous enzymatically addressable materials have been explored for a variety of applications such as payload delivery [42] , diagnostic monitoring [43] and ligand presentation [44] , [45] , [46] . Although much effort has been focused on understanding the biological function of endogenous IDPs, our study suggests that these proteins represent an untapped resource for biomaterial design. IDPs could contribute to the development of new biosynthetic coatings, fusion proteins whose functions may be sterically gated and novel cell surface engineering strategies. As described earlier, IDPs may be designed de novo , synthesized at high purity, and chemically tailored at specific positions along the chain through mutagenesis. IDP sequences can be optimized for specific applications through directed-evolution approaches and synthesized to include bio-orthogonal chemical moieties via the use of unnatural amino acids. Indeed, IDPs based on nucleoporin proteins have recently been incorporated into synthetic gated pores [47] and surface-grafted layers [48] , supporting the idea that IDPs can be manipulated in ways that are analogous to synthetic polymers. Together with these efforts, our work hints at the value of exploring IDPs as a new class of ‘smart’ biomaterial building blocks. Cloning and expression of rNFH-SA Expression vectors were constructed by modifying the multiple cloning site of pET6 × HN-C (Clontech Inc.) to include the EcoR1 and HindIII restriction enzyme recognition sequences. The modified expression vector was digested with EcoR1 and HindIII and subsequently purified. A HindIII restriction enzyme site was introduced at the end of NFH-SA gene cloned in pCIneo by site-directed mutagenesis [49] . The modified NFH-SA gene was excised from the pCIneo vector by EcoR1 and HindIII digestion, ligated to the linearized, modified pET6 × HN-C vector, and transformed into competent Escherichia coli cells. Plasmids isolated from the resulting transformants were screened by a diagnostic restriction enzyme digestion and sequenced. The expression vector was transformed into the E. coli Rosetta strain (Novagen) for expression. Confluent starter cultures (grown overnight) were transferred to expression cultures and incubated with shaking at 37 °C. Expression was induced by the addition of isopropyl β-D-1-thiogalactopyranoside to a final concentration of 0.75 mM. The cells were typically harvested 3 h after induction by centrifugation at 3,000 g for 20 min at 4 °C. Purification of rNFH-SA The cell pellet was resuspended in 20 mM Tris pH 8.0, 300 mM NaCl, 1 mM tris(2-carboxyethyl)phosphine hydrochloride (TCEP), 1 mM phenylmethanesulfonylfluoride and lysed by sonic disruption at 4 °C. The cell lysate was centrifuged at 20,000 g for 15 min at 4 °C to remove insoluble cellular matter and then applied to a nickel-nitrilotriacetic acid affinity column. After subsequent washes with increasing concentration of imidazole, the purified protein was eluted using 200 mM imidazole. Ion exchange chromatography using a linear elution gradient of increasing ionic strength over a diethylaminoethyl cellulose anion exchange resin was used as a polishing step to improve purity when needed. Circular dichroism CD spectra were recorded from 250 to 190 nm on a Jasco-720 spectropolarimeter. Spectra were obtained using a cuvette with a 1-mm path length at 25 °C at a bandwidth of 1 nm with a scanning rate of 10 nm s −1 in continuous scanning mode and a response time of 5 s. The collected raw spectra were buffer subtracted and converted from millidegrees to molar ellipticity as described elsewhere [50] . To study the protein under different solution conditions, the protein was desalted into distilled water, lyophilized and then re-dissolved in the appropriate pH/ionic strength solution. Appropriate controls were included to ensure that desalting and lyophilization did not introduce conformational changes. The solutions used in this study include water at pH 2.4, 6.3 and 10.9, and water with 50 mM NaCl at pH 2.4 and 10.9. Dynamic light scattering Dynamic light scattering experiments were performed on a Dynapro Nanostar (Wyatt Technology, Santa Barbara, CA, USA) operating at 658 nm. Measurements were performed at room temperature (25 °C) in triplicates, in 20 mM Tris pH 8.0, 1 mM TCEP. All data were analyzed using a dedicated software package (Dynamics, version 7.1, Wyatt Technology). To study the effect of different solution conditions, the protein solution was prepared as described for CD. Functionalization of silica and quartz surfaces Functionalization of silica coverslips for AFM, quartz substrates for QCM-D experiments and silicon substrates for ellipsometry were carried out as described previously [51] . Substrates were activated via plasma cleaning prior to functionalization. After rinsing with water and drying in a nitrogen stream, the surfaces were subsequently silanized with glycidyloxypropyltrimethoxysilane (GOPTS) for 45 min at 75 °C. The surfaces were then rinsed with acetone and reacted with diamino-polyethylene glycol (molecular weight of 400 Da) for 4 h at 75 °C. After rinsing with water and drying in a nitrogen stream, the surface amines were reacted with a saturated solution of 3-(Maleimido)propionic acid N-hydroxysuccinimide ester (NHS-maleimide) in dry dimethylformamide for 45 min at room temperature to yield maleimide-functionalized surfaces. This sequence of reactions is shown in Supplementary Fig. 3 . Substrates for AFM and ellipsometry experiments were subsequently incubated under a 5 mg ml −1 solution of rNFH-SA in phosphate buffered saline (PBS) for 20 h followed by rinsing in PBS. Quartz crystal microbalance with dissipation QCM-D measurements were performed with a Q-Sense E4 system. Quartz crystals with fundamental frequencies of ~5 MHz were functionalized as described in the previous section and used for immobilization of rNFH-SA. Either 0.5 or 5 mg ml −1 of the rNFH-SA solution was prepared in PBS at pH 7.5 and injected into the flow cell with a rate of typically 50 μl min −1 , using a syringe pump. Change in frequency ( Δf ) and dissipation ( ΔD ) were measured at five overtones ( n =3, 5 … 11) simultaneously. After an initial binding was observed, the pump was turned off and the protein was incubated on the surface for either 4 h (0.5 mg ml −1 ) or 20 h (5 mg ml −1 ) depending on the protein concentration. The adsorbed protein on the crystal was then washed with buffer to remove any non-specifically bound material. The data were fit using the Voight–Voinova model [21] for viscoelastic films to obtain the mass of the hydrated protein layer bound to the surface. Spectroscopic ellipsometry Silicon wafers (UniversityWafer, Inc.) were cut into 1 cm 2 pieces for use as SE substrates. The substrates were functionalized as described in the previous section. SE measurements were conducted on an alpha-SE system (J.A. Woollam Co., Inc.) at an angle of incidence of 70° in the spectral range of 380 to 890 nm under air at room temperature. Data was collected on surfaces functionalized with the NHS-maleimide cross-linker to model the underlying surface chemistry consisting of GOPTS, diamino-polyethylene glycol and the cross-linker. The height and refractive index obtained from this analysis was then used to model the data collected on surfaces functionalized with the rNFH-SA. Ellipsometric data were modelled using the CompleteEASE software as described in Supplementary Note 2 . Atomic force microscopy Force measurements were made using a Molecular Force Probe three-dimensional instrument (MFP, Asylum Research, Inc.). The experimental setup uses an open cell arrangement with a wetted tip brought into contact with the wetted sample surface. Silicon nitride cantilevers (OTR4-10) calibrated using the thermal method built into the MFP with a nominal spring constant of 0.02 N m −1 were used. The tips had a radius of curvature of <20 nm. Force curves were typically collected over 500 nm with at least 2,048 data points per curve, at a rate of 1 Hz. Relative triggers of up to 4 nN were used to prevent the tip from damaging the surface. When exchanging solutions of different ionic strength, both the sample and tip were rinsed with several millilitres of the new solution prior to a measurement. At least 400 force curves were recorded for each sample at different points on the surface. The brush height was measured as the tip–sample separation at which the force began to increase from zero. Briefly, the raw AFM data (deflection error versus sensor displacement) was converted to force–distance curves (force versus tip–sample separation) as described by Cappella et al. [52] The contact region was fit to a straight line and the point of hard contact was identified. The force profile at large separation was averaged to a baseline value, and the tip-sample separation at the first point where the force deviated significantly (at least three times the s.d. of the baseline fit) from the baseline value was denoted as the brush height. All of the above procedures were performed in MATLAB. Protease digestion The protein brush was incubated either with thrombin (1 U μl −1 , GE Healthcare) or clostripain (43 U ml −1 , Worthington Biochemicals). Thrombin was prepared in PBS pH 7.4 and clostripain was prepared in its activation buffer containing 25 mM phosphate, 1 mM calcium acetate and 2.5 mM dithiothreitol. The surface was spotted in triplicates with both 1 and 0.5 μl of enzyme and allowed to incubate overnight at room temperature. A 1 μl spot of both buffer and bovine serum albumin (1 mg ml −1 ) were included as controls. The surface was stained with a primary antibody targeted towards the HN tag on rNFH-SA and the appropriate fluorescent secondary antibody. The surface was imaged using a Typhoon scanner to obtain fluorescence images. For AFM experiments, the surface was prepared with 3 μl spots each of the enzyme, corresponding buffer and water at pH 10.9. The surface was washed after overnight incubation and all subsequent measurements were performed in water at pH 10.9. The height measured on the water-incubated spot (data not shown) functioned as a control to ensure that incubation in the buffer did not affect the brush height. How to cite this article : Srinivasan, N. et al. Stimuli-sensitive intrinsically disordered protein brushes. Nat. Commun. 5:5145 doi: 10.1038/ncomms6145 (2014).